The atypical mechanosensitive microRNA-712 derived from pre-ribosomal RNA induces endothelial inflammation and atherosclerosis MicroRNAs (miRNAs) regulate cardiovascular biology and disease, but the role of flow-sensitive microRNAs in atherosclerosis is still unclear. Here we identify miRNA-712 (miR-712) as a mechanosensitive miRNA upregulated by disturbed flow ( d-flow ) in endothelial cells, in vitro and in vivo. We also show that miR-712 is derived from an unexpected source, pre-ribosomal RNA, in an exoribonuclease-dependent but DiGeorge syndrome critical region 8 (DGCR8)-independent manner, suggesting that it is an atypical miRNA. Mechanistically, d-flow -induced miR-712 downregulates tissue inhibitor of metalloproteinase 3 (TIMP3) expression, which in turn activates the downstream matrix metalloproteinases (MMPs) and a disintegrin and metalloproteases (ADAMs) and stimulate pro-atherogenic responses, endothelial inflammation and permeability. Furthermore, silencing miR-712 by anti-miR-712 rescues TIMP3 expression and prevents atherosclerosis in murine models of atherosclerosis. Finally, we report that human miR-205 shares the same ‘seed sequence’ as murine-specific miR-712 and also targets TIMP3 in a flow-dependent manner. Targeting these mechanosensitive ‘athero-miRs’ may provide a new treatment paradigm in atherosclerosis. Atherosclerosis is the major underlying cause of cardiovascular pathologies and preferentially occurs in arterial regions exposed to disturbed flow ( d-flow ) by altering the gene expression [1] , [2] , [3] , [4] . Vascular endothelial cells respond to blood flow through mechanosensors that transduce the mechanical force associated with flow (known as shear stress) into cell signalling events and changes in gene expression [5] , [6] , [7] . D-flow and stable flow ( s-flow) promotes and inhibits atherogenesis, respectively, in large part by regulating discrete sets of pro-atherogenic and atheroprotective genes [1] , [8] , [9] . While s-flow upregulates atheroprotective genes such as Klf2, Klf4 and eNOS , d-flow upregulates a number of pro-atherogenic genes including vascular cell adhesion molecule-1 ( VCAM-1 ) [1] , [10] and matrix metalloproteinases ( MMPs ) [11] , which mediate pro-angiogenic, pro-inflammatory, proliferative and pro-apoptotic responses, promoting atherosclerosis [5] , [12] , [13] . The ways in which the mechanosensitive machinery in endothelial cells regulates gene expression and contributes to these pro-atherogenic events is still poorly understood, especially in the in vivo setting. MicroRNAs (miRNAs) are small non-coding RNA molecules that modulate the stability and/or the translational efficiency of their target messenger RNAs. miRNAs have been demonstrated to be involved in key physiological and pathophysiological aspects of cardiovascular biology but the role of flow-sensitive miRNAs in atherosclerosis is still unclear. To address this knowledge gap, we recently developed a mouse model of flow-induced atherosclerosis by partially ligating the left carotid artery (LCA) of the ApoE −/− mouse [10] . This model directly demonstrates the causal relationship between d-flow and atherosclerosis as the LCA rapidly develops robust atherosclerosis within 2 weeks following partial ligation that causes d-flow with characteristic low and oscillatory shear stress (OS), while the contralateral, undisturbed right common carotid artery (RCA) remains healthy [10] ( Fig. 1a ). In addition, we developed a method of isolating intimal RNA from mouse carotid artery following ligation [1] , [10] . This method allows easy and rapid endothelial-enriched RNA isolation that is virtually free of contamination from the vascular smooth muscle cells (VSMCs) and leukocytes. Using this mouse model and the RNA isolation method, we identified more than 500 mechanosensitive genes, including novel ones such as lmo4 , klk10 and dhh , and confirming well-known mechanosensitive genes, such as VCAM-1, klf2 and eNOS 1 . In this study, we used this model to identify mechanosensitive miRNAs regulated by d-flow and their role in endothelial inflammation and atherosclerosis. 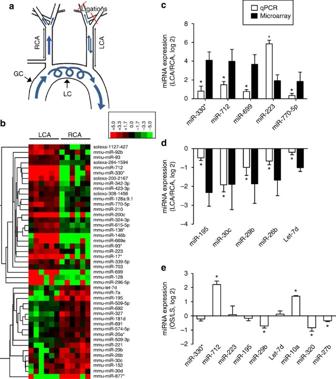Figure 1: miR-712 is a flow-sensitive miRNA upregulated byd-flow in vitroandin vivo. (a) The schema shows naturally occurringd-flow(lesser curvature, LC) ands-flowregions (greater curvature, GC) in the aortic arch. Also shown is the surgically inducedd-flowin partial carotid ligation model in which three of the four caudal branches of the left common carotid artery (LCA) are ligated, while the contralateral right common carotid artery (RCA) remains untouched as an internal control. (b) Endothelial-enriched total RNAs obtained from intima of mouse (C57BL/6) left carotid (flow-disturbed LCA) and right carotid (contralateral control, RCA) at 48 h post ligation were analysed by gene array (Illumina BeadChip). Hierarchical clustering analyses of mechanosensitive miRNAs found in LCA endothelium compared with that of RCA are shown as heat maps. The colour represents the expression level of the gene. Red represents high expression, while green represents low expression. The expression levels are continuously mapped on the colour scale provided at the top of the figure. Each column represents a single sample pooled from three different LCAs or RCAs, and each row represents a single miRNA probe (n=3). (c–f) Validation of miRNA microarray results by qPCR. Quantitative PCR (qPCR), using additional independent RNA samples, was used to validate the above miRNA array data. Ten miRNAs (five up-, five downregulated miRNAs at 48 h post ligation) were selected based on fold change by flow. The qPCR study validated the microarray results for (c) five upregulated (miR-712, -330*, -699, -223 and 770-5p) and (d) five downregulated (miR-195, -30c, -29b, -26b and let-7d) miRNAs at the 48 h time point (n=5 each, data shown as mean±s.e.m.; *P<0.05 as determined by pairedt-test). To further validate whether the mechanosensitive miRNAs that were identifiedin vivoresponded specifically to shear stress, we tested expression of these miRNAsin vitrousing iMAECs that were subjected to LS or OS, mimickings-flowandd-flow in vitro, respectively14. Among the nine different miRNAs examined, seven miRNAs were differentially expressed under OS (n=6 each, data shown as mean±s.e.m.; *P<0.05 as determined by pairedt-test) (e). These results showed that miR-712 was the most consistently and robustly upregulated miRNA bothin vivoand under d-flow conditionsin vitro. Figure 1: miR-712 is a flow-sensitive miRNA upregulated by d-flow in vitro and in vivo. ( a ) The schema shows naturally occurring d-flow (lesser curvature, LC) and s-flow regions (greater curvature, GC) in the aortic arch. Also shown is the surgically induced d-flow in partial carotid ligation model in which three of the four caudal branches of the left common carotid artery (LCA) are ligated, while the contralateral right common carotid artery (RCA) remains untouched as an internal control. ( b ) Endothelial-enriched total RNAs obtained from intima of mouse (C57BL/6) left carotid (flow-disturbed LCA) and right carotid (contralateral control, RCA) at 48 h post ligation were analysed by gene array (Illumina BeadChip). Hierarchical clustering analyses of mechanosensitive miRNAs found in LCA endothelium compared with that of RCA are shown as heat maps. The colour represents the expression level of the gene. Red represents high expression, while green represents low expression. The expression levels are continuously mapped on the colour scale provided at the top of the figure. Each column represents a single sample pooled from three different LCAs or RCAs, and each row represents a single miRNA probe ( n =3). ( c – f ) Validation of miRNA microarray results by qPCR. Quantitative PCR (qPCR), using additional independent RNA samples, was used to validate the above miRNA array data. Ten miRNAs (five up-, five downregulated miRNAs at 48 h post ligation) were selected based on fold change by flow. The qPCR study validated the microarray results for ( c ) five upregulated (miR-712, -330*, -699, -223 and 770-5p) and ( d ) five downregulated (miR-195, -30c, -29b, -26b and let-7d) miRNAs at the 48 h time point ( n =5 each, data shown as mean±s.e.m. ; * P <0.05 as determined by paired t- test). To further validate whether the mechanosensitive miRNAs that were identified in vivo responded specifically to shear stress, we tested expression of these miRNAs in vitro using iMAECs that were subjected to LS or OS, mimicking s-flow and d-flow in vitro , respectively [14] . Among the nine different miRNAs examined, seven miRNAs were differentially expressed under OS ( n =6 each, data shown as mean±s.e.m. ; * P <0.05 as determined by paired t- test) ( e ). These results showed that miR-712 was the most consistently and robustly upregulated miRNA both in vivo and under d-flow conditions in vitro. Full size image Here we identify miRNA-712 (miR-712) as the most flow-sensitive miRNA that is upregulated by d-flow in endothelial cells, in vivo and in vitro . We also identified a novel miRNA biogenesis mechanism from RN45S gene in a non-canonical manner. Further studies identify tissue inhibitor of metalloproteinase 3 (TIMP3) as a direct target of miR-712, which induces endothelial inflammation and atherosclerosis. Treatment with specific antagonist of miR-712 (anti-miR-712) inhibits endothelial inflammation, barrier function and atherosclerosis in a TIMP3-dependent manner in mouse models of atherosclerosis. Collectively, our results suggest that targeting the mechanosensitive miRNAs by their anti-miRs may provide a novel potential therapeutic approach to treat atherosclerosis. miR-712 is a flow-sensitive miRNA upregulated by d-flow To identify mechanosensitive miRNAs in arterial endothelium in vivo , we carried out miRNA array analyses using endothelial-enriched RNAs from partially ligated mouse carotids ( Fig. 1a ) as in our prior analyses of mechanosensitive mRNAs [1] and integrated these two genome-wide data sets using a systems biology approach to help us identify relevant miRNA-target gene connections. The in vivo microarray data showed that 45 (27 up- and 18 downregulated) miRNAs were altered by more than 50% in the LCA endothelium compared with the RCA at 12 and 48 h post ligation ( Fig. 1b , and Supplementary Fig. S1a and Supplementary Table S1 ). Quantitative PCR (qPCR) using additional independent RNA samples was used to validate the miRNA array data for the top 10 most mechanosensitive miRNAs (5 up-, 5 downregulated miRNAs at 48 h post ligation): upregulated (miR-330*, 712, 699, 223 and 770-5p) and downregulated (miR-195, 30c, 29b, 26b and let-7d) miRNAs ( Fig. 1c,d ; Supplementary Fig. S1b ). To determine whether these mechanosensitive miRNAs that were identified in vivo responded specifically to shear stress, we tested expression of these miRNAs in vitro using immortalized mouse aortic endothelial cells (iMAECs) that were subjected to laminar shear (LS) or OS, mimicking s-flow and d-flow in vitro , respectively [14] ( Fig. 1e ). These results showed that miR-712 was the most consistently and robustly upregulated miRNA both in vivo and under flow conditions in vitro , leading us to further characterize its expression and function. A time course study showed that miR-712 was upregulated significantly in the d-flow region (LCA) compared with s-flow region (RCA) at 48 h post ligation in mouse carotids ( Fig. 2a ). Using the miScript qPCR assay that can distinguish between the pre-miR and mature forms of miR-712, we found that pre-miR-712 expression significantly increased at 48 h post ligation, while expression of mature miR-712 increased significantly in LCA at 24 and 48 h post partial ligation ( Fig. 2b,c ), which was subsequently validated by sequencing the PCR amplicons (data not shown). This suggests that d-flow initially stimulate processing of pre-existing miR-712 precursor form into the mature form within 24 h, which is then followed by biogenesis of pre-miR-712 and its concurrent processing to the mature form later on, in mouse artery in vivo . 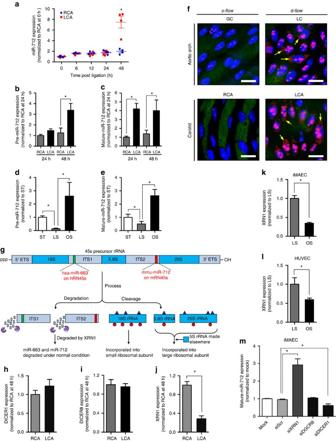Figure 2: miR-712 is atypically derived fromRN45Sgene in XRN1-dependent manner. (a) Expression of miR-712 was determined by qPCR using endothelial-enriched RNA obtained from LCA and RCA following partial carotid ligation in C57Bl6 mouse (0–48 h) (n=4, data shown as mean±s.e.m.; *P<0.05 as determined by pairedt-test). (b,c) Expression of pre-miR-712 and mature miR-712 byd-flowin LCA and RCA endothelium following partial ligation at 24 and 48 h as above inawas quantitated by miScript miRNA qPCR assay (n=8 each; *P<0.05 as determined by Student’st-test). (d,e) Expression of pre-miR-712 and mature miR-712 was measured by miScript miRNA qPCR in iMAECs exposed to laminar (LS), oscillatory shear (OS) or static (ST) for 24 h (n=6, data shown as mean±s.e.m.; *P<0.05 as determined by Student’st-test). (f) Aortic arch (LC and GC) and LCA and RCA obtained at 2 days post ligation from C57Bl6 mice were subjected to fluorescencein situhybridization using DIG-labelled miR-712 probe and anti-DIG antibody, which was detected by tyramide signal amplification method using Cy3 and confocal microscopy (shown in red), (n=6). Blue: DAPI nuclear stain; green: autofluorescent elastic lamina; arrows indicate cytosolic miR-712 expression. White scale bars, 20 μm. Panelgshows the potential structure and processing of pre-ribosomal RNA gene,RN45s, which is composed of 18S, 5.8S and 28S rRNA sequences with two intervening spacers ITS1 and ITS2. The sequences matching murine miR-712 in ITS2 and its putative human counterpart miR-663 in ITS1 are indicated as well. (h–j) Expression ofDICER,DGCR8andXRN1in mouse RCA and LCA (2 days post ligation) was determined by qPCR (n=4, data shown as mean±s.e.m.; *P<0.05 as determined by pairedt-test). (k,l)XRN1expression in iMAECs and HUVECs exposed to LS or OS for 24 h was determined by qPCR (n=3 each, data shown as mean±s.e.m.; *P<0.05 as determined by Student’st-test). (m) miR-712 expression was induced by treating iMAECs with XRN1 siRNA but not by DGCR8 siRNA and DICER1 siRNA (n=3 each, data shown as mean±s.e.m.; *P<0.05 as determined by Student’st-test). Figure 2: miR-712 is atypically derived from RN45S gene in XRN1-dependent manner. ( a ) Expression of miR-712 was determined by qPCR using endothelial-enriched RNA obtained from LCA and RCA following partial carotid ligation in C57Bl6 mouse (0–48 h) ( n =4, data shown as mean±s.e.m. ; * P <0.05 as determined by paired t- test). ( b , c ) Expression of pre-miR-712 and mature miR-712 by d-flow in LCA and RCA endothelium following partial ligation at 24 and 48 h as above in a was quantitated by miScript miRNA qPCR assay ( n= 8 each; * P <0.05 as determined by Student’s t- test). ( d , e ) Expression of pre-miR-712 and mature miR-712 was measured by miScript miRNA qPCR in iMAECs exposed to laminar (LS), oscillatory shear (OS) or static (ST) for 24 h ( n =6, data shown as mean±s.e.m. ; * P <0.05 as determined by Student’s t- test). ( f ) Aortic arch (LC and GC) and LCA and RCA obtained at 2 days post ligation from C57Bl6 mice were subjected to fluorescence in situ hybridization using DIG-labelled miR-712 probe and anti-DIG antibody, which was detected by tyramide signal amplification method using Cy3 and confocal microscopy (shown in red), ( n =6). Blue: DAPI nuclear stain; green: autofluorescent elastic lamina; arrows indicate cytosolic miR-712 expression. White scale bars, 20 μm. Panel g shows the potential structure and processing of pre-ribosomal RNA gene, RN45s , which is composed of 18S, 5.8S and 28S rRNA sequences with two intervening spacers ITS1 and ITS2. The sequences matching murine miR-712 in ITS2 and its putative human counterpart miR-663 in ITS1 are indicated as well. ( h – j ) Expression of DICER , DGCR8 and XRN1 in mouse RCA and LCA (2 days post ligation) was determined by qPCR ( n =4, data shown as mean±s.e.m. ; * P <0.05 as determined by paired t- test). ( k , l ) XRN1 expression in iMAECs and HUVECs exposed to LS or OS for 24 h was determined by qPCR ( n =3 each, data shown as mean±s.e.m. ; * P <0.05 as determined by Student’s t- test). ( m ) miR-712 expression was induced by treating iMAECs with XRN1 siRNA but not by DGCR8 siRNA and DICER1 siRNA ( n =3 each, data shown as mean±s.e.m. ; * P <0.05 as determined by Student’s t- test). Full size image Exposure of iMAECs to OS for 24 h in vitro also dramatically increased the expression of mature and precursor forms of miR-712 compared with LS as determined by qPCR ( Fig. 2d,e ) and northern blot ( Supplementary Fig. S2 ), confirming the flow sensitivity of miR-712. Studies using in situ hybridization with a miR-712 probe (Exiqon) showed significantly increased expression of miR-712 in the LCA endothelium, compared with the RCA ( Fig. 2f , lower panel), further validating the in vivo microarray and qPCR results. To rule out whether increased expression of miR-712 in LCA was not simply due to an acute change in mechanical environment created by the partial ligation surgery, we tested the expression of miR-712 in mouse aortic arch where the atherosclerosis-prone lesser curvature (LC) and athero-protected greater curvature (GC) are naturally and chronically exposed to d-flow and s-flow , respectively ( Fig. 1a ). Expression of miR-712 was significantly higher in the flow-disturbed LC compared with GC ( Fig. 2f , upper panel; Supplementary Fig. S3 ). This result was further corroborated by qPCR assay using endothelial-enriched RNA obtained from the LC and GC regions of aortic arch ( Supplementary Fig. S4 ). Interestingly, we also found that miR-712 expression was increased in the plasma of mice that underwent partial carotid ligation but not in shams ( Supplementary Fig. S5 ). These findings suggest that miR-712 is indeed a flow-sensitive miRNA, which is significantly upregulated in endothelial cells exposed to d-flow in the aortic arch naturally or in LCA on partial carotid ligation, as well as in vitro. miR-712 is generated from RN45S gene in an atypical manner The genomic locus and biogenesis pathway of miR-712 were not known. Our nucleotide sequence search revealed that the pre-miR-712 sequence matched to the internal transcribed spacer 2 (ITS2) region of the murine pre-ribosomal RNA, RN45s gene ( Fig. 2g ), which is still not completely annotated. The RN45S encodes for 45S, which contains sequences for 18, 5.8 and 28S rRNAs along with two intervening spacers, ITS1 and ITS2 ( Fig. 2g ). Since ribosomal RNAs have never been reported to be a source of miRNAs, we examined whether miR-712 biogenesis was regulated by the canonical pathway using the DiGeorge syndrome critical region 8 (DGCR8)/DROSHA and DICER miRNA processors [15] , [16] , [17] or by non-canonical pathways [18] , [19] in a flow-dependent manner. Expression of DICER1 and DGCR8 was not altered by flow in endothelial cells in vitro (iMAEC) and in vivo (mouse carotids and aortic arch) ( Fig. 2h,i , Supplementary Fig. S6a,b ). Since XRN1 is an exonuclease that is known to degrade the ITS2 region during the processing of RN45S (ref. 20 ), we tested whether XRN1 is shear dependent and regulates biogenesis of miR-712. We found that XRN1 expression was downregulated by d-flow in the mouse carotid ( Fig. 2j ) and aortic arch ( Supplementary Fig. S6c ) and in human and mouse endothelial cells in vitro ( Fig. 2k,l ). Further, knockdown of XRN1 by short interfering RNA (siRNA) treatment increased the expression of miR-712, suggesting that reduction of XRN1 under d-flow conditions led to accumulation of miR-712 ( Fig. 2m and Supplementary Figs S6d and S7a ). In contrast, knockdown of the canonical miRNA processor DGCR8 did not affect miR-712 expression ( Fig. 2m and Supplementary Figs S6e and S7 ). These results suggest that miR-712 is a murine-specific, non-canonical miRNA derived from an unexpected source, pre-ribosomal RNA, in a XRN1-dependent, but DGCR8-independent and DICER1-dependent manner. To test whether this novel mechanism of miRNA biogenesis from pre-ribosomal RNA exists in humans as well, we examined human RN45S gene for putative miRNAs using a computational prediction program, miREval [21] , [22] . This search revealed that human-specific miR-663 could be derived from RN45s gene ( Fig. 2g ) in addition to its previously annotated genomic locus on chromosome 2 (miRBase). Interestingly, like miR-712, miR-663 was previously identified from a microarray study as one of the most shear-sensitive miRNAs in human endothelial cells and was shown to induce endothelial inflammation, a key atherogenic step [14] , raising a possibility that they share a common biogenesis pathway and roles in endothelial function. Consistent with this hypothesis, we found that XRN1 expression is inhibited by OS ( Fig. 2l ) and that siRNA knockdown of XRN1 significantly increased miR-663 expression in human endothelial cells ( Supplementary Fig. S6f,g ). miR-712 targets TIMP3 in the endothelium Through in silico analyses using miR-712-predicted target gene list from TargetScan and the mechanosensitive gene list using the same mouse model [1] , we identified TIMP3 as a potential gene target. TIMP3 was selected for further study since the miR-712 interactome analysis ( Fig. 3a ; Supplementary Fig. S8 ) suggested its potential role as a key gene hub connected to numerous genes of interest, including MMP2/9 and a disintegrin and metalloproteinase 10/17 ( ADAM10/17 ), ADAM with thrombospondin type 1 motif, 4 ( ADAMTS4 ) and versican that are known to play a critical role in the regulation of vascular inflammation, permeability and atherosclerosis [23] , [24] , [25] , [26] , [27] , [28] . 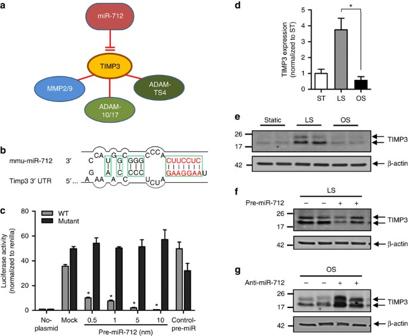Figure 3: TIMP3 is the direct target of miR-712. Panelashows TIMP3 as a potential target of miR-712 and its link to putative downstream metalloproteinase targets. Panelbshows the seed sequence of miR-712 and complementary 3′-UTR sequence of TIMP3. (c) iMAECs transfected with dual-luciferase reporter plasmids containing wild-type (WT) or mutant TIMP3-3′-UTR were treated with pre-miR-712 or control pre-miR. Firefly luciferase activity (normalized to controlRenillaluciferase) indicating TIMP3 expression was determined using Luc-Pair miR Luciferase Assay Kit (n=3 each, data shown as mean±s.e.m.; *P<0.05 as determined by Student’st-test). (d)TIMP3expression in iMAECs determined by qPCR was decreased by exposure to OS compared with LS or ST for 24 h (n=6, data shown as mean±s.e.m.; *P<0.05 as determined by Student’st-test). (e–g) Representative western blots show modulation of TIMP3 expression by shear stress in the presence of pre-miR-712 or anti-miR-712 for 24 h in iMAECs. (e) TIMP3 expression decreased by OS compared with LS for 24 h. (f) Treatment with pre-miR-712 (20 nM) downregulated TIMP3 expression under LS condition. (g) anti-miR-712 (400 nM) treatment rescued OS-induced loss of TIMP3. β-actin was used as an internal loading control. Full sized scans of all western blots are provided inSupplementary Figs S19 and S20. Figure 3: TIMP3 is the direct target of miR-712. Panel a shows TIMP3 as a potential target of miR-712 and its link to putative downstream metalloproteinase targets. Panel b shows the seed sequence of miR-712 and complementary 3′-UTR sequence of TIMP3. ( c ) iMAECs transfected with dual-luciferase reporter plasmids containing wild-type (WT) or mutant TIMP3-3′-UTR were treated with pre-miR-712 or control pre-miR. Firefly luciferase activity (normalized to control Renilla luciferase) indicating TIMP3 expression was determined using Luc-Pair miR Luciferase Assay Kit ( n =3 each, data shown as mean±s.e.m. ; * P <0.05 as determined by Student’s t- test). ( d ) TIMP3 expression in iMAECs determined by qPCR was decreased by exposure to OS compared with LS or ST for 24 h ( n =6, data shown as mean±s.e.m. ; * P <0.05 as determined by Student’s t- test). ( e – g ) Representative western blots show modulation of TIMP3 expression by shear stress in the presence of pre-miR-712 or anti-miR-712 for 24 h in iMAECs. ( e ) TIMP3 expression decreased by OS compared with LS for 24 h. ( f ) Treatment with pre-miR-712 (20 nM) downregulated TIMP3 expression under LS condition. ( g ) anti-miR-712 (400 nM) treatment rescued OS-induced loss of TIMP3. β-actin was used as an internal loading control. Full sized scans of all western blots are provided in Supplementary Figs S19 and S20 . Full size image To test whether miR-712 targets TIMP3 in endothelial cells ( Fig. 3b ), we employed a dual-luciferase reporter assay in iMAECs transfected with either wild-type or mutated TIMP3 3′-UTR firefly luciferase constructs. Treatment of cells with pre-miR-712 inhibited luciferase activity in a dose-dependent manner, while mutant or control pre-miR had no effect ( Fig. 3c ), demonstrating that miR-712 binds to the TIMP3 3′-UTR and inhibits its expression in endothelial cells. Next, we tested whether TIMP3 expression was regulated by flow in a miR-712-dependent manner. Exposure of iMAECs to OS for 24 h significantly decreased TIMP3 mRNA and protein expression, compared with LS ( Fig. 3d,e ). Pre-miR-712 treatment decreased expression of TIMP3 in LS-exposed cells ( Fig. 3f ), while inhibition of miR-712 using locked nucleic acid (LNA)-based anti-miR-712 increased TIMP3 expression in cells exposed to OS ( Fig. 3g ). These findings demonstrate that miR-712 upregulated by OS is directly responsible for the loss of TIMP3 expression in endothelial cells. To examine the biological relevance of reduced TIMP3 by miR-712, we tested tumour necrosis factor α (TNFα)-converting enzyme (TACE/ADAM17) activity by measuring soluble-TNFα released into the conditioned medium by treating cells with pre-miR-712 versus anti-miR-712 or siTIMP3 versus TIMP3 overexpression vector in iMAECs under static or shear conditions. We found that soluble TNFα release into the conditioned medium was increased by OS ( Fig. 4a ), which was inhibited by anti-miR-712 treatment or TIMP3 overexpression ( Fig. 4b ; Supplementary Fig. S9 ). In contrast, pre-miR-712 treatment or TIMP3 knockdown increased release of soluble TNFα into the conditioned media in static and LS-exposed cells ( Fig. 4b ; Supplementary Fig. S9 ). These results suggest that ADAM17/TACE activity was regulated by OS in a miR-712- and TIMP3-dependent manner. In addition, endothelial inflammation was increased by pre-miR-712 as measured by monocyte (J774.1 cells) adhesion to endothelium ( Fig. 4c ). Furthermore, endothelial permeability as determined in iMAECs using by fluorescent dextran was also increased by pre-miR-712, which was inhibited by the overexpression of TIMP3 ( Fig. 4d ). Taken together, these results indicate that mechanistically TIMP3 is downstream of miR-712 and inhibition of miR-712 by anti-miR-712 treatment or overexpression of TIMP3 can overcome endothelial inflammation induced by d-flow . 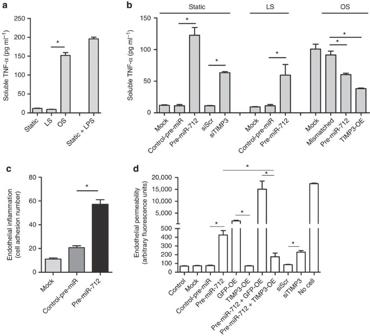Figure 4: miR-712 induces endothelial inflammation and hyperpermeability changes. (a) iMAECs were exposed to static, LS or OS for 24 h, and the conditioned media were used for TNFα enzyme-linked immunosorbent assay (ELISA). LPS was used as a positive control. (b) iMAECs were transfected with TIMP3 expression vector (TIMP3-OE), TIMP3 siRNA (150 nM), pre-miR-712 (20 nM), anti-miR-712 (400 nM) and respective controls for 24 h. Cells were then exposed to static, LS or OS for 24 h, and s-TNFα in conditioned media was determined by ELISA. (n=6, data shown as mean±s.e.m.; *P<0.05 as determined by one-way analysis of variance (ANOVA)). (c) iMAECs were transfected with pre-miR-712 (20 nM) or control and leukocyte adhesion assay was performed using 2.5 × 105fluorescent-labelled J774.4 mouse monocyte cells. Adherent cells were counted (n=5 independent experiments, data shown as mean±s.e.m.; *P<0.05 as determined by one-way ANOVA). (d) iMAECs were transfected with TIMP3-OE or its GFP vector control (GFP-OE), TIMP3 or scrambled control siRNA (siTIMP3 or siScr, 150 nM), pre-miR-712 or control pre-miR (20 nM), pre-miR-712 with GFP-OE or TIMP3-OE, and no treatment (control), transfection (mock) or no cell controls for 24 h. Cells were then exposed to static, LS or OS for 24 h, and endothelial permeability was determined using a FITC-dextran-basedin vitrovascular permeability kit (Cultrex). Fluorescence signals from FITC-dextran in the lower chamber were quantified and plotted as arbitrary fluorescence units (n=3 each from two independent experiments, data shown as mean±s.e.m.; *P<0.05 as determined by one-way ANOVA). Figure 4: miR-712 induces endothelial inflammation and hyperpermeability changes. ( a ) iMAECs were exposed to static, LS or OS for 24 h, and the conditioned media were used for TNFα enzyme-linked immunosorbent assay (ELISA). LPS was used as a positive control. ( b ) iMAECs were transfected with TIMP3 expression vector (TIMP3-OE), TIMP3 siRNA (150 nM), pre-miR-712 (20 nM), anti-miR-712 (400 nM) and respective controls for 24 h. Cells were then exposed to static, LS or OS for 24 h, and s-TNFα in conditioned media was determined by ELISA. ( n =6, data shown as mean±s.e.m. ; * P <0.05 as determined by one-way analysis of variance (ANOVA)). ( c ) iMAECs were transfected with pre-miR-712 (20 nM) or control and leukocyte adhesion assay was performed using 2.5 × 10 5 fluorescent-labelled J774.4 mouse monocyte cells. Adherent cells were counted ( n =5 independent experiments, data shown as mean±s.e.m. ; * P <0.05 as determined by one-way ANOVA). ( d ) iMAECs were transfected with TIMP3-OE or its GFP vector control (GFP-OE), TIMP3 or scrambled control siRNA (siTIMP3 or siScr, 150 nM), pre-miR-712 or control pre-miR (20 nM), pre-miR-712 with GFP-OE or TIMP3-OE, and no treatment (control), transfection (mock) or no cell controls for 24 h. Cells were then exposed to static, LS or OS for 24 h, and endothelial permeability was determined using a FITC-dextran-based in vitro vascular permeability kit (Cultrex). Fluorescence signals from FITC-dextran in the lower chamber were quantified and plotted as arbitrary fluorescence units ( n =3 each from two independent experiments, data shown as mean±s.e.m. ; * P <0.05 as determined by one-way ANOVA). Full size image In vivo delivery of anti-miR-712 to mouse endothelium To test whether d-flow -induced miR-712 plays a key role in atherosclerosis, mice were treated with LNA-based anti-miR-712. First, we found that anti-miRs can be effectively delivered to arterial endothelium in vivo as demonstrated by two independent methods: confocal en face imaging of TexasRed-labelled control LNA-anti-miR ( Fig. 5a and Supplementary Fig. S10a–d ) and autoradiography of 64 Cu-labelled anti-miR-712 ( Fig. 5b and Supplementary Fig. S10e,f ). Interestingly, both fluorescent-labelled anti-miR and radiolabelled anti-miR preferentially accumulated in the flow-disturbed LCA and aortic arch, which is probably due to increased endothelial mass transfer [29] and permeability to macromolecules in d-flow areas [30] . A dose-curve study showed that anti-miR-712 (5 mg kg −1 , subcutaneously (s.c.)) effectively silenced d-flow -induced miR-712 expression in LCA endothelium as compared with the mismatched control ( Fig. 5c ), and this dose was used for all subsequent studies. We found that the expression of TIMP3 mRNA and protein was reduced in d-flow regions both in the partially ligated LCA and aortic arch LC compared with RCA and GC, respectively, and it was rescued by the anti-miR-712 treatment ( Fig. 5d and Supplementary Fig. S11 ). This further demonstrates the role of miR-712 in regulation of TIMP3 expression in a flow-dependent manner in vivo . Since TIMP3 is a well-known inhibitor of MMPs and ADAMs, we examined the effect of anti-miR-712 on these metalloproteinase activities in vivo . MMP activity ( in situ zymography) and ADAMs activity (versican cleavage by immunohistochemical staining) were increased by d-flow in LCA compared with RCA that were significantly blunted by anti-miR-712 treatment ( Fig. 5e,f ). Further, anti-miR-712 treatment inhibited vascular hyperpermeability and junctional vascular endothelial (VE)-cadherin decrease induced by d-flow in partially ligated LCA in mouse ( Supplementary Fig. S12 ). These in vivo results, taken together with the in vitro findings shown above, provide strong evidence for a direct hierarchical link between d-flow , miR-712, TIMP3 and its downstream metalloproteinase activity, and endothelial inflammation and barrier dysfunction in arterial wall, which are well-known pro-atherogenic events. 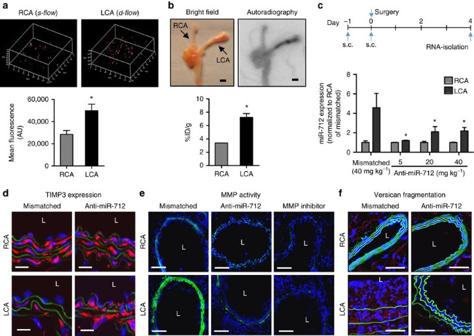Figure 5: Anti-miR-712 silences miR-712 and restores TIMP3 expressionin vivo. (a) TexRed-615-labelled control anti-miR or saline was injected (s.c.) in C57Bl6 mice. Carotid arteries were dissected out 24 h later, and using Zeiss 510 confocal microscope z-stack images of theen facesections were obtained. Images were rendered to three dimensions, bounding box was drawn on the area of interest and scaled coordinate axes were drawn and fluorescence signals from Red channel were processed and quantified. Graph shows mean fluorescence intensity of TexRed-615 signals from carotids (n=5, data shown as mean±s.e.m.). (b) Following partial carotid ligation and HFD for 2 weeks, ApoE−/−mice were injected with64Cu-labelled anti-miR-712 via tail vein. After 3 h, aortic trees including carotids were prepared and autoradiographed, which was used to quantitate percentage of injected dose per gram (n=6, data shown as mean±s.e.m.; *P<0.05 as determined by Student’st-test). Scale bar, 1 mm. (c) To determine the optimal dose of anti-miR-712, C57Bl6 mice were injected with anti-miR-712 daily for 2 days (s.c. at 5, 20 or 40 mg kg−1per day) and followed by partial carotid ligation. Mismatched anti-miR-712 (40 mg kg−1per day) was used as a control. Endothelial-enriched RNAs were prepared from LCA and RCA obtained at 4 days post ligation, and miR-712 expression was determined by qPCR showing optimal effect at 5 mg kg−1dose (n=4 each, data shown as mean±s.e.m.; *P<0.05 as determined by pairedt-test). (d–f) ApoE−/−mice were partially ligated and fed HFD for 1 week (d,e) or 2 weeks (f). RCA and LCA frozen sections obtained from these mice were used for immunofluorescence staining with antibody specific to TIMP3 shown in red (scale bar, 20 μm) (d) or versican fragment peptide DPEAAE shown in red (scale bar, 20 μm) (f), andin situzymography using DQ-gelatin (green) to determine MMP activity (e). As a control for the MMP activity assay, some LCA and RCA sections were incubated with MMP inhibitor 1. Blue: DAPI and green: autofluorescent elastic lamina (L=lumen of the artery). Scale bar, 50 μm. Figure 5: Anti-miR-712 silences miR-712 and restores TIMP3 expression in vivo. ( a ) TexRed-615-labelled control anti-miR or saline was injected (s.c.) in C57Bl6 mice. Carotid arteries were dissected out 24 h later, and using Zeiss 510 confocal microscope z-stack images of the en face sections were obtained. Images were rendered to three dimensions, bounding box was drawn on the area of interest and scaled coordinate axes were drawn and fluorescence signals from Red channel were processed and quantified. Graph shows mean fluorescence intensity of TexRed-615 signals from carotids ( n =5, data shown as mean±s.e.m.). ( b ) Following partial carotid ligation and HFD for 2 weeks, ApoE −/− mice were injected with 64 Cu-labelled anti-miR-712 via tail vein. After 3 h, aortic trees including carotids were prepared and autoradiographed, which was used to quantitate percentage of injected dose per gram ( n =6, data shown as mean±s.e.m. ; * P <0.05 as determined by Student’s t- test). Scale bar, 1 mm. ( c ) To determine the optimal dose of anti-miR-712, C57Bl6 mice were injected with anti-miR-712 daily for 2 days (s.c. at 5, 20 or 40 mg kg −1 per day) and followed by partial carotid ligation. Mismatched anti-miR-712 (40 mg kg −1 per day) was used as a control. Endothelial-enriched RNAs were prepared from LCA and RCA obtained at 4 days post ligation, and miR-712 expression was determined by qPCR showing optimal effect at 5 mg kg −1 dose ( n =4 each, data shown as mean±s.e.m. ; * P <0.05 as determined by paired t- test). ( d – f ) ApoE −/− mice were partially ligated and fed HFD for 1 week ( d , e ) or 2 weeks ( f ). RCA and LCA frozen sections obtained from these mice were used for immunofluorescence staining with antibody specific to TIMP3 shown in red (scale bar, 20 μm) ( d ) or versican fragment peptide DPEAAE shown in red (scale bar, 20 μm) ( f ), and in situ zymography using DQ-gelatin (green) to determine MMP activity ( e ). As a control for the MMP activity assay, some LCA and RCA sections were incubated with MMP inhibitor 1. Blue: DAPI and green: autofluorescent elastic lamina (L=lumen of the artery). Scale bar, 50 μm. Full size image Anti-miR-712 treatment decreases atherosclerotic lesions Finally, we tested the role of miR-712 in two different models of atherosclerosis using ApoE −/− mice: the partial carotid ligation model fed a high-fat diet (HFD) that rapidly develops atherosclerosis within 2 weeks [10] and the conventional western diet-fed model that chronically develops atherosclerosis in 3 months [31] . In the carotid ligation model, the LCA rapidly developed atherosclerosis within 2 weeks ( Fig. 6a ) and treatment with anti-miR-712 (5 mg kg −1 , s.c. twice a week for 2 weeks) significantly reduced atherosclerosis lesion development and immune cell infiltration compared with the mismatched-anti-miR-712 or saline controls ( Fig. 6a–e ). Similarly, anti-miR-712 treatment (5 mg kg −1 , s.c. twice a week for 3 months) significantly inhibited atherosclerosis development in the conventional western diet model in whole aortas as well as in the aortic arch ( Fig. 6f–i ). In both models, anti-miR-712 did not affect the serum lipid profile ( Supplementary Table S2 ). These findings demonstrate a potent inhibitory effect of anti-miR-712 in two different murine models of atherosclerosis. In addition, we found that tail vein injection of recombinant adenoviral TIMP3 (AdTIMP3) significantly increased the expression of TIMP3 in aorta and in blood cells ( Supplementary Fig. S13 ) and inhibited atherosclerotic lesion development in the partial carotid ligation model ( Fig. 6j,k ). 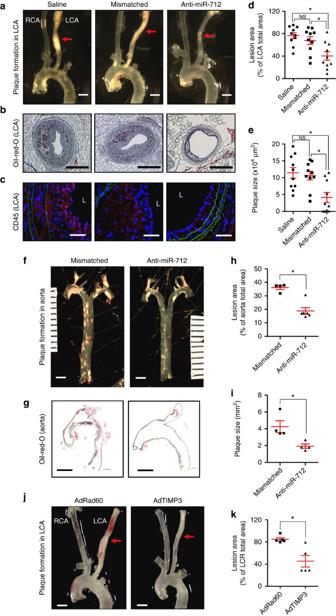Figure 6: Anti-miR-712 or AdTIMP3 reduces atherosclerosis in ApoE−/−mice. For acute study,ApoE−/−mice were pretreated twice with anti-miR-712 or mismatched control (5 mg kg−1each, s.c.) or saline on 1 and 2 days before partial ligation. Mice were then fed a HFD and anti-miR and control treatments were continued (twice a week s.c.) for 2 weeks. (a) Aortic trees including the carotids were dissected and examined by bright field imaging and lesion area was quantified ind(n=10 each, data shown as mean±s.e.m.; *P<0.05 as determined by one-way analysis of variance (ANOVA)). Scale bar, 1 mm. (b) Frozen sections prepared from the middle parts of these arteries, denoted by red arrows inawere stained with Oil-Red-O and plaque size was quantified ine(n=10 each, data shown as mean±s.e.m.; *P<0.05 as determined by one-way ANOVA). Scale bar, 200 μm. (c) Representative confocal imaging of frozen sections immunostained with CD45 antibody is shown (n=10). Scale bar, 20 μm. For chronic study,ApoE−/−mice were fed western diet (without any partial ligation surgery) and were treated with anti-miR-712 (5 mg kg−1, twice a week, s.c.) or mismatched control for 3 months (n=10 each). (f) Aortic trees were dissected and examined byen faceOil-Red-O staining and the lesion area was quantified inh(n=4–6 in each group, data shown as mean±s.e.m.; *P<0.05 as determined by Student’st-test). Scale bar, 2 mm. Some aortic arches were longitudinally sectioned and stained with Oil-Red-O (g) and plaque size was quantified ini(n=4 each, data shown as mean±s.e.m.; *P<0.05 as determined by Student’st-test). Scale bar, 2 mm. (j) For TIMP3 overexpression,ApoE−/−mice were injected once with AdTIMP3 (108p.f.u. per animal, via tail vein) or control virus (RAD60, 108p.f.u. per animal) 5 days before partial carotid ligation and high-fat diet for 2 weeks. (j) Aortic trees including the carotids were dissected and examined by bright field imaging and lesion area was quantified ink(n=5, data shown as mean±s.e.m.; *P<0.05 as determined by Student’st-test). Scale bar, 1 mm. Figure 6: Anti-miR-712 or AdTIMP3 reduces atherosclerosis in ApoE −/− mice. For acute study, ApoE −/− mice were pretreated twice with anti-miR-712 or mismatched control (5 mg kg −1 each, s.c.) or saline on 1 and 2 days before partial ligation. Mice were then fed a HFD and anti-miR and control treatments were continued (twice a week s.c.) for 2 weeks. ( a ) Aortic trees including the carotids were dissected and examined by bright field imaging and lesion area was quantified in d ( n =10 each, data shown as mean±s.e.m. ; * P <0.05 as determined by one-way analysis of variance (ANOVA)). Scale bar, 1 mm. ( b ) Frozen sections prepared from the middle parts of these arteries, denoted by red arrows in a were stained with Oil-Red-O and plaque size was quantified in e ( n =10 each, data shown as mean±s.e.m. ; * P <0.05 as determined by one-way ANOVA). Scale bar, 200 μm. ( c ) Representative confocal imaging of frozen sections immunostained with CD45 antibody is shown ( n =10). Scale bar, 20 μm. For chronic study, ApoE −/− mice were fed western diet (without any partial ligation surgery) and were treated with anti-miR-712 (5 mg kg −1 , twice a week, s.c.) or mismatched control for 3 months ( n =10 each). ( f ) Aortic trees were dissected and examined by en face Oil-Red-O staining and the lesion area was quantified in h ( n =4–6 in each group, data shown as mean±s.e.m. ; * P <0.05 as determined by Student’s t- test). Scale bar, 2 mm. Some aortic arches were longitudinally sectioned and stained with Oil-Red-O ( g ) and plaque size was quantified in i ( n =4 each, data shown as mean±s.e.m. ; * P <0.05 as determined by Student’s t- test). Scale bar, 2 mm. ( j ) For TIMP3 overexpression, ApoE −/− mice were injected once with AdTIMP3 (10 8 p.f.u. per animal, via tail vein) or control virus (RAD60, 10 8 p.f.u. per animal) 5 days before partial carotid ligation and high-fat diet for 2 weeks. ( j ) Aortic trees including the carotids were dissected and examined by bright field imaging and lesion area was quantified in k ( n =5, data shown as mean±s.e.m. ; * P <0.05 as determined by Student’s t- test). Scale bar, 1 mm. Full size image Since anti-miR-712 was delivered via s.c. injection to mice in our study, anti-miR-712 could affect other tissues and cell types in addition to our primary target, arterial endothelial cells. We found that anti-miR-712 treatment downregulated the miR-712 expression in multiple tissues, including whole blood and spleen ( Supplementary Fig. S14 ). Of note, anti-miR-712 treatment significantly inhibited miR-712 expression in blood ( Supplementary Fig. S14a ), which was shown to be increased following partial carotid ligation surgery, but not in sham controls ( Supplementary Fig. S5 ). Also, in the arterial wall, expression of miR-712 increased in media and adventitia of the LCA ( Supplementary Fig. S15 ). To determine whether miR-712 plays an important role in the media, we performed smooth muscle cell migration and proliferation assays and found that miR-712 stimulated VSMC migration, but not proliferation ( Supplementary Fig. S16 ). Taken together, these findings suggest that miR-712 produced in LCA endothelium could be transferred to circulation and adjacent medial smooth muscle cells, contributing to additive pro-atherogenic effects. The miR-205 is a potential human homologue of murine mir-712 Since miR-712 is a murine-specific miRNA, we searched whether there are any miR-712 homologues in humans. Using short sequence nucleotide alignment and search tool (BLAST, http://www.blast.ncbi.nlm.nih.gov ), we found that miR-205 shares the same ‘seed sequence’ with miR-712 and is highly conserved in most vertebrates including humans and mice ( Fig. 7a ). In addition, miR-205 and miR-712 share more than 50% of the putative targets (including TIMP3) as shown by the TargetScan analysis ( Fig. 7b ). Importantly, like miR-712, we found that miR-205 expression (both precursor and mature forms) is higher in iMAECs and human aortic endothelial cells exposed to OS than that of LS ( Fig. 7c,d ). In addition, miR-205 expression was higher in mouse LCA (endothelium as well as media and adventitia) compared with the RCA at 48 h post partial ligation ( Fig. 7e ). To validate whether miR-205 targets TIMP3, we treated iMAECs and human aortic endothelial cells (HAECs) with pre-miR-205 and found that miR-205 downregulates TIMP3 in a concentration-dependent manner ( Fig. 7f,g ). Collectively, these findings suggest that miR-205 shares the seed sequence with miR-712, is also a flow-sensitive miRNA, and targets TIMP3, suggesting that miR-205 is a potential human homologue of murine miR-712. 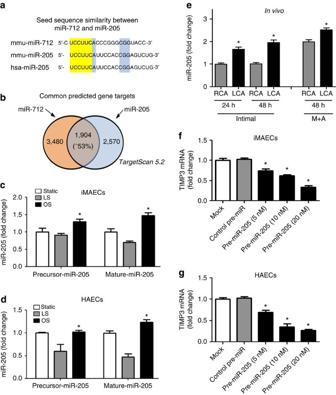Figure 7: miR-205 is a flow-sensitive human homologue of murine miR-712. (a) The highlighted region in yellow shows the seed sequence match between the murine miR-712 and murine and human miR-205, and those shown in blue indicate additional conserved sequences. (b) The putative targets of miR-712 and miR-205 obtained from TargetScan were compared. Venn diagram depicts the common gene targets of miR-205 and miR-712. (c) Expression of precursor and mature miR-205 in iMAECs exposed to static, LS or OS for 24 h (n=4; data shown as means±s.e.m.; *P<0.05 as determined by Student’st-test). (d) Expression of precursor and mature miR-205 in human aortic endothelial cells (HAECs) exposed to static, LS or OS for 24 h (n=4; data shown as means±s.e.m.; *P<0.05 as determined by Student’st-test). (e) Expression of mature miR-205 was determined using the RNAs obtained from the endothelial-enriched (intimal region) and the leftover medial and adventitia region (M+A) of the LCA and RCA at 24 and 48 h post partial ligation, respectively. Expression ofTIMP3was determined by qPCR in (f) iMAECs and (g) HAECs transfected with increasing concentrations of pre-miR-205 or control pre-miR compared with vehicle controls (mock) (n=3; data shown as means±s.e.m.; *P<0.05 as determined by Student’st-test). Figure 7: miR-205 is a flow-sensitive human homologue of murine miR-712. ( a ) The highlighted region in yellow shows the seed sequence match between the murine miR-712 and murine and human miR-205, and those shown in blue indicate additional conserved sequences. ( b ) The putative targets of miR-712 and miR-205 obtained from TargetScan were compared. Venn diagram depicts the common gene targets of miR-205 and miR-712. ( c ) Expression of precursor and mature miR-205 in iMAECs exposed to static, LS or OS for 24 h ( n =4; data shown as means±s.e.m. ; * P <0.05 as determined by Student’s t -test). ( d ) Expression of precursor and mature miR-205 in human aortic endothelial cells (HAECs) exposed to static, LS or OS for 24 h ( n =4; data shown as means±s.e.m. ; * P <0.05 as determined by Student’s t -test). ( e ) Expression of mature miR-205 was determined using the RNAs obtained from the endothelial-enriched (intimal region) and the leftover medial and adventitia region (M+A) of the LCA and RCA at 24 and 48 h post partial ligation, respectively. Expression of TIMP3 was determined by qPCR in ( f ) iMAECs and ( g ) HAECs transfected with increasing concentrations of pre-miR-205 or control pre-miR compared with vehicle controls (mock) ( n =3; data shown as means±s.e.m. ; * P <0.05 as determined by Student’s t -test). Full size image Collectively, our results demonstrate that miR-712 is an atypical mechanosensitive miRNA originating from the RN45S gene and regulates endothelial inflammation and barrier function by targeting TIMP3. We also showed that anti-miR-712 treatment in vivo can effectively silence miR-712 expression in arterial endothelial cells, restoring TIMP3 levels and inhibiting atherosclerotic plaque development in two different murine models of atherosclerosis. The identification of miR-712 as a flow-dependent miRNA was based on our in vivo miRNA microarray study that was carried out using the endothelial-enriched RNA directly from the surgically induced d-flow regions of mouse carotid arteries. Endothelial samples from the LC region of aortic arch, where they are naturally and chronically exposed to d-flow , also showed increased expression of miR-712, demonstrating that the miR-712 induction in the LCA is not a mere surgical artifact. Further, miR-712 expression was increased in endothelial cells exposed to OS compared with LS, demonstrating its shear sensitivity. Together, these results demonstrate that miR-712 is flow-sensitive miRNA in endothelial cells, both in vivo and in vitro. Here we identified the genomic locus of miR-712 in RN45S gene and its atypical biogenesis mechanism. miR-712 is a murine-specific miRNA and its sequence turns out to be derived from the ITS2 region of mouse RN45S gene. Similarly, we identified that human-specific miR-663 could be derived from the spacer region of human RN45S gene as well. Interestingly, these spacer regions of ribosomal RNA contain species-specific nucleotide sequences that are used as phylogenetic markers [32] . In addition, following the transcription of rRNAs, these spacer regions are rapidly degraded by XRN1 exonuclease [33] . Our data showed that d-flow decreased the expression of XRN1 but not the canonical miRNA processors DGCR8/DROSHA in both human and mouse endothelial cells, indicating that there may be a common role of XRN1 in human miR-663 and murine miR-712. Indeed, knockdown of XRN1 significantly increased miR-712 and miR-663 expression while knockdown of DGCR8 did not. These results indicate that miR-712 induction by d-flow is dependent on XRN1 but independent of the canonical miRNA processors. This suggests that the novel miRNA biogenesis mechanism using RN45S gene in the XRN1-dependent manner may not be exclusive to murine and human species. It is intriguing that both murine miR-712 and human miR-663 were identified as the most mechanosensitive miRNAs that were upregulated by d-flow from two completely independent array studies [14] . These results further support the hypothesis that murine miR-712 and human miR-663 are derived from their respective RN45S genes by a common mechanism involving XRN1 and may serve as pro-atherogenic miRNAs. In this study, we showed how spacer regions of ribosomal RNA can serve as the precursor material for the miRNAs and how knockdown of XRN1 can lead to increased synthesis of the miR-712 in mouse and miR-663 in humans under d-flow conditions. To the best of our knowledge, this is the first report demonstrating that miRNAs can be derived from the spacer regions of the rRNAs. Whether XRN1 is directly or indirectly responsible for biogenesis of these atypical miRNAs needs to be further studied. Here we showed that miR-712 directly downregulates the expression of TIMP3. This is consistent with previous observations that TIMP3 is frequently downregulated in atherosclerosis [34] . TIMP3 is a key hub gene that regulates inflammation, barrier function and extracellular matrix remodelling by inhibiting multiple metalloproteinases such as MMP2/9, ADAM10, ADAMTS4 and ADAM17/TACE that are well-established players in atherosclerosis [34] . Our study showed that miR-712 downregulates TIMP3 under d-flow conditions leading to activation of MMP2/9 and ADAM activities. MMP2/9 activity was remarkably increased in the LCA, which was significantly inhibited by anti-miR-712 treatment. The ADAM-family proteases are known to cleave the extracellular matrix proteoglycans such as versican, which is known to induce pro-atherogenic responses including endothelial inflammation [35] . We found increased versican fragmentation by d-flow in LCA, which was inhibited by anti-miR-712 treatment. In addition, d-flow increased endothelial permeability in a manner dependent on miR-712 and TIMP3, which is likely to be mediated by ADAMs such as ADAM17/TACE. ADAM17, which is also known as TACE, induces shedding of membrane-bound TNFα and VE-cadherin leading to soluble-TNFα release and destabilization of junctional integrity [36] . Consistent with this idea, we found that d-flow increased soluble-TNFα release in vitro , increased endothelial permeability and decreased junctional VE-cadherin expression in LCA ( Supplementary Fig. S12 ), which were significantly reversed by anti-miR-712 treatment. Collectively, these findings demonstrate a potent role of miR-712-TIMP3-MMP/ADAM axis induced by d-flow on regulation of endothelial inflammation and permeability in the arterial wall. Since TIMP3 is not likely to be the sole target of miR-712, we attempted to identify additional miR-712 targets in endothelium. We used in silico analyses ( Supplementary Fig. S8 ), low-density qPCR array of candidate genes and proteomics approach to identify additional miR-712 targets. Unfortunately, in this study, we were unable to validate additional flow-dependent miR-712 targets in endothelial cells. While our results do not rule out the possibility of other target genes, our findings clearly demonstrate the critical role of TIMP3 as the major miR-712 target regulating endothelial inflammation and atherosclerosis. Several mechanosensitive miRNAs have been identified in endothelial cells but their role in atherosclerosis is still unclear. LS stimulates the expression of miR-10a, miR-19a, miR-21, miR-23b, miR-101 and miR-143/145, mediating anti-atherogenic events [37] , [38] , [39] , [40] , [41] , [42] , while OS induces the expression of miR-21, miR-92a and miR-663 leading to pro-atherogenic responses [14] , [43] , [44] . miR-155 is also flow-sensitive miRNA but its role in atherosclerosis is controversial [45] . Here we provide evidence that miR-712 is an important mechanosensitive miRNA that is highly upregulated by d-flow and plays a critical role in atherosclerosis by affecting endothelial inflammation and barrier function. Using two different murine models of atherosclerosis, we showed that anti-miR-712 treatment prevents atherosclerosis by effectively silencing miR-712 expression, thereby restoring TIMP3 activity. We also demonstrated the inhibitory effect of AdTIMP3 on atherosclerosis in partially ligated ApoE −/− mice, further substantiating the role of TIMP3 in flow-induced atherosclerosis. One caveat of this study is that anti-miR-712 was systemically delivered to mice and, therefore, it is likely to affect multiple tissues and cell types in addition to our primary target (arterial endothelial cells). Indeed, anti-miR-712 treatment silenced miR-712 expression in multiple tissues, including whole blood and spleen ( Supplementary Fig. S14 ). Previously, miR-143/145 produced in endothelial cells were shown to be transferred to smooth muscle cells [46] . Consistent with this, miR-712 expression increased in media and adventitia of the LCA ( Supplementary Fig. S15 ). Moreover, we found that miR-712 expression was increased in blood following partial carotid ligation surgery but not in sham controls and anti-miR-712 treatment inhibited it ( Supplementary Figs S5 and S14a ). We speculate that miR-712 produced in endothelial cells under d-flow conditions can be transferred to smooth muscle cells and blood where it may have functional impact leading to robust atherosclerosis. Since miR-712 is a murine-specific miRNA, its therapeutic value in human atherosclerosis could be limited. In this study, however, we identified miR-205 as a human homologue of the murine miR-712. It is unclear why our initial microarray study did not show statistically significant change in miR-205 expression in the LCA compared with RCA. One possibility is an inherent limitations in the miRNA array probe design [47] . However, using specific qPCR probes for precursor and mature miR-205, we found that miR-205 is flow sensitive, like miR-712, in endothelial cells both in vitro and in vivo. We also showed that miR-205 shares the same seed sequence with miR-712 and is highly conserved in most vertebrates including humans and mice ( Fig. 7a ) and targets TIMP3. Therefore, knowledge gained from the miR-712 study could be translatable to humans, providing a potential clinical relevance. In conclusion, we identified a mechanism by which mechanosensitive miR-712 can be generated from the pre-ribosomal RNA gene in an XRN1-dependent, but DGCR8-independent and DICER1-dependent manner, providing novel evidence that flow-sensitive miRNAs could be derived from an unexpected yet abundant source, pre-ribosomal RNAs. In addition, we demonstrate that anti-miRs targeting mechanosensitive miRNAs could be used to inhibit atherosclerosis. Our findings clearly demonstrate TIMP3 as a major target of miR-712 that controls endothelial inflammation and atherosclerosis. We propose that d-flow reduces the expression of XRN1, which increases miR-712 expression derived from the pre-ribosomal RNA ( Fig. 8 ). Increased miR-712 downregulates TIMP3 expression, which in turn activates MMPs and ADAM proteases, leading to endothelial inflammation, hyperpermeability and arterial wall matrix fragmentation. miR-712 may also be transferred to blood and arterial medial layer where it may affect leukocytes and VSMC migration, respectively, resulting in multitude of pro-atherogenic changes ( Fig. 8 ). Targeting these mechanosensitive ‘athero-miRs’ such as miR-712 and miR-205 may provide a new treatment paradigm in atherosclerosis. 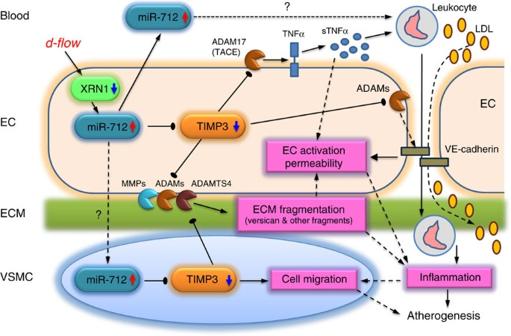Figure 8: Summary and working hypothesis. miR-712 induces inflammation and atherosclerosis by targeting TIMP3.D-flowstimulates miR-712 expression in endothelium by an XRN1-dependent mechanism. Increased miR-712 stimulates endothelial inflammation, permeability and extracellular matrix (ECM) fragmentation by downregulating TIMP3, which is a critical inhibitor of matrix metalloproteinases (MMPs and ADAMs). Decreased TIMP3 expression by miR-712 induces inflammation and atherosclerosis by activating a multitude of metalloproteinases: (1) ADAM17/TACE that releases soluble-TNFα that may induce local and systemic inflammation; (2) ADAMs that shed junctional VE-cadherin, increasing permeability that facilitates LDL and leukocyte infiltration; (3) ADAMTS leading to versican fragmentation; and (4) MMPs leading to ECM degradation leading to vessel wall remodeling. In addition, miR-712 expression is also increased in whole blood and vascular smooth muscle cells (VSMCs) suggesting either transfer of miR-712 from endothelium to these compartments or increase in its local production in these compartments. Increased miR-712 in VSMCs induces their migration while circulating miR-712 may affect blood leukocytes further contributing to atherogenesis. Figure 8: Summary and working hypothesis. miR-712 induces inflammation and atherosclerosis by targeting TIMP3. D-flow stimulates miR-712 expression in endothelium by an XRN1-dependent mechanism. Increased miR-712 stimulates endothelial inflammation, permeability and extracellular matrix (ECM) fragmentation by downregulating TIMP3, which is a critical inhibitor of matrix metalloproteinases (MMPs and ADAMs). Decreased TIMP3 expression by miR-712 induces inflammation and atherosclerosis by activating a multitude of metalloproteinases: (1) ADAM17/TACE that releases soluble-TNFα that may induce local and systemic inflammation; (2) ADAMs that shed junctional VE-cadherin, increasing permeability that facilitates LDL and leukocyte infiltration; (3) ADAMTS leading to versican fragmentation; and (4) MMPs leading to ECM degradation leading to vessel wall remodeling. In addition, miR-712 expression is also increased in whole blood and vascular smooth muscle cells (VSMCs) suggesting either transfer of miR-712 from endothelium to these compartments or increase in its local production in these compartments. Increased miR-712 in VSMCs induces their migration while circulating miR-712 may affect blood leukocytes further contributing to atherogenesis. Full size image Mouse partial carotid ligation surgery All animal procedures were approved by the Animal Care and Use Committees at Emory University and University of California at Davis. Male C57BL/6 and ApoE −/− mice (Jackson Laboratory, Bar Harbor) were fed ad libitum with standard chow diet until surgery at 8–9 weeks of age. Mice were anaesthetized with 3.5% isoflurane initially and then 1.5–2% during the entire procedure and underwent partial ligation [10] . The LCA bifurcation was exposed by blunt dissection and three of four caudal LCA branches (left external carotid, internal carotid and occipital arteries) were ligated with 6-0 silk sutures, leaving the superior thyroid artery intact. The contralateral RCA was left intact as an internal control. Following surgery, analgesic buprenorphine (0.1 mg kg −1 ) was administrated. Two different models of atherosclerosis using ApoE −/− mice were used: the partial carotid ligation model fed a Paigen’s HFD (Science Diets) containing 1.25% cholesterol, 15% fat and 0.5% cholic acid [1] and the Western diet-fed model for 3 months [31] . Ultrasonography Following carotid ligation, d-flow in LCA was confirmed by Doppler ultrasonography (Vevo770, Visualsonics) with a 30-MHz probe. Briefly, mice were anaesthetized with 2% isoflurane and body temperature was monitored with a rectal probe and regulated by use of a heating pad. First, using B-mode, a long axis view of RCA and LCA was obtained. Thereafter, during diastole, a short-axis view was taken to visualize each artery [10] , [48] . LNA-based anti-miR treatment or AdTIMP3 injection in vivo LNA-based miRNA inhibitor (anti-miR-712, Exiqon) were administered s.c. to 8-week-old male mice. For delivery efficiency testing, C57BL/6 mice ( n=3 ) were s.c. administrated with 5 mg kg −1 of Texas-Red-615-labelled anti-miR control (TEX615/5′-ACGTCTATACGCCCA-3′) or saline. After 24 h, aortas were excised and tissue samples were mounted on glass slides after counterstaining with 4′,6-diamidino-2-phenylindole (DAPI, Sigma). Samples were imaged using a Zeiss LSM 510 META confocal microscope (Carl Zeiss). To study the inhibition of miR-712, LNA-based anti-miR-712 (5′-GTACCGCCCGGGTGAAGGA-3′) or mismatched control was s.c. administered to C57BL/6 mice ( n=4 ) 1 day before and on the day of partial ligation surgery. Animals were killed on the fourth day post ligation and the carotid intimal RNAs were extracted and expression of miR-712 was determined by qPCR. For TIMP3 treatment, replication-defective recombinant adenoviruses encoding for TIMP3 (AdTIMP3) or empty vector control (AdRAD60) were used [49] . ApoE −/− mice were injected once with AdTIMP3 (10 8 p.f.u. per animal, via tail vein) or control virus (AdRAD60, 10 8 p.f.u. per animal) 5 days before partial carotid ligation and high-fat diet for 2 weeks. For atherosclerosis studies, aortic trees were dissected out and processed for immunohistochemical analysis, and plaque analysis was done using NIH Image J [10] . Synthesis of anti-miR-712-DOTA The conjugation of 5′-modified anti-miR-712 (5′-/5AmMC6/+CGCCCGGGTGAAGA‐3′, Exiqon, and DOTA-NHS-ester (1,4,7,10-tetraazacyclododecane-1,4,7,10-tetraacetic acid mono ( N -hydroxysuccinimide ester), Macrocyclics) followed a previously published paper [50] with modifications. A 5′-modified anti-miR-712 (0.19 μmol, 1 mg) was suspended in 0.2 M borated buffer (0.3 ml, pH 8.5) and the dimethylsulphoxide solution (20 μl, Aldrich) of DOTA-NHS-ester (3.6 μmol, 2.8 mg) was added. After 5 h of reaction, the mixture of DOTA-conjugated anti-miR-712 was purified on Sephadex G-25 filled with double-distilled water. Isolated anti-miR-712-DOTA was purified by HPLC with the following conditions: column Clarity Oligo-PR (250 × 10.00 mm 2 , 5 μ, Phenomenex), gradient-solvent B (5–30%, 0–30 min, solvent A-0.1 M triethylammonium acetate, solvent B-acetonitrile). Collected fractions were concentrated by centrifugation with an Amicon Ultra-4 centrifugal filter unit (molecular weight cutoff: 3k). The concentrated solution was lyophilized and anti-miR-712-DOTA was stored at −20 °C. Mass spectrometric analysis of sample was performed with Thermo Fisher Scientific LTQ Orbitrap (San Jose, CA) operated in the centroid mode ( Supplementary Fig. S17 ). The deconvoluted mass from 1,413.43 ( Z =4) was detected at 5,657.7 g mol −1 (Calc. molecular weight=5,657.6). Radiolabeling of anti-miR-712-DOTA 64 CuCl 2 was obtained from Washington University Medical School under a protocol controlled by the University of California, Davis. 64 CuCl 2 (3–5 mCi) was added into 0.1 M ammonium citrate buffer (0.1 ml, pH 5.5) and the anti-miR-712-DOTA (1 mM, 3–4 μl) in double-distilled water was slowly added. After incubation for 1 h at 40 °C, the pH was adjusted to 7 by 1 M sodium hydroxide solution (trace metal, Aldrich). The reaction mixture was aspirated into 5 ml triethylammonium acetate (10 mM, pH 7.0–7.5) in a 10-ml syringe. The solution was eluted through a Sep-Pak light C18 cartridge (Waters, Milford, MA). The C18 cartridge was eluted by 95% methanol (0.5–0.8 ml) to release the radiolabelled product. Concentrated solution was diluted with PBS to prepare a dose of ~0.2–0.3 mCi per 150 μl. The specific activity of 64 Cu-anti-miR-712-DOTA was ~500–750 mCi μmol −1 . Radiochemical purity measured by a binary pump HPLC system (Waters) was more than 95% ( Supplementary Fig. S18 ). Animal biodistribution and autoradiography studies 64 Cu-labelled anti-miR-712-DOTA was administered by tail vein injection of 2–3 μg (0.2–0.3 mCi) in PBS (1 × , 150 μl each animal). After 3 h, animals were killed by intraperitoneal injection of Euthasol (Western Medical Supply), blood and urine samples were collected, and the body was perfused with DMEM (Invitrogen) to remove blood, and organs were collected. The aorta including the right and left carotid arteries were dissected and placed on a phosphor screen (Amersham Biosciences) for 1 h. The phosphor screen was scanned on a Storm-860 imaging system (Amersham Biosciences) with 50 μm resolution. Radioactivity was counted with a 1,470 automatic gamma counter (PerkinElmer). Tissue samples were weighed on a microbalance and the biodistribution is reported as percent injected radioactivity per gram of tissue. Serum lipid analysis Serum lipid analysis was performed commercially (Cardiovascular Specialty Laboratories, Atlanta, GA) using a Beckman CX7 biochemical analyser and reagents from Beckman Diagnostics (Fullerton, CA) for total cholesterol, triglycerides, HDL and LDL [51] . Plaque lesion analysis Aorta and carotid arteries were isolated en bloc as described above from ligated ApoE −/− mice fed a HFD for 2 weeks. RCA and LCA were photographed using a charge-coupled device camera (Moticam 2500, Motic) attached to a dissection microscope (EMZ-8TRD, MEIJI Techno) at × 3 magnification and the opaque area covered by plaque and total artery area of LCA were quantified using NIH ImageJ software [1] . miRNA microarray procedures and data analysis Intimal RNAs from three LCAs or RCAs were pooled to obtain ~30 ng total RNA [10] . miRNA microarray was performed using Illumina Mouse v2 MicroRNA expression BeadChip array (Illumina) at the Emory Biomarker Service Center [14] . After hybridization, BeadChips were scanned on the Illumina BeadArray Reader to determine probe fluorescence intensity and the raw probe intensities were normalized using the quantile normalization algorithm [1] . The normalized microarray data were statistically analysed using Significance Analysis of Microarrays software (SAM 3.0) [1] . The differentially expressed miRNAs between LCA and RCA were identified for those that showed more than 1.5-fold changes at less than 10% false discovery rate. Quantitative real-time PCR Total RNA was polyadenylated and reverse transcribed for use in a two-step quantitative reverse transcribed–PCR using the NCode miRNA First-Strand cDNA Synthesis and qRT-PCR kits (Invitrogen). The resulting complementary DNA was subjected to qPCR using the NCode universal reverse primer in conjunction with a sequence-specific forward primer for selected miRNAs. Small nucleolar RNA 202 (Sno202) and U6B were used as the internal control using ABI StepOne Plus qPCR machine. The PCR conditions were 10 min at 95 °C, followed by 40 cycles of 95 °C for 4 s and 60 °C for 30 s. For measurement of mRNA targets, qPCR was performed on selected genes using Brilliant II SYBR Green QPCR Master Mix (Stratagene) with custom designed primers using 18S as house-keeping control [1] . Fold changes between LCA and RCA were determined for all targets using the ΔΔCt method [1] . Sequences for primers used for miRNA expression and mRNA expression studies have been listed in Supplementary Tables S3 and S4 , respectively. Mature and precursor miRNA assays were performed using miRNA quantification and was performed by SYBR green qPCR assay using miScript reverse transcription kit (Qiagen) according to the manufacturer’s instructions. qPCR was performed using miScript SYBR Green PCR kit (Qiagen) with miScript universal primer (U6B) and the miRNA-specific forward primers and relative fold change was calculated [1] . The specific mature and pre-miR primers were purchased from Qiagen. Other primer sequences used for microarray validation were designed based on the miRNA sequences obtained from the miRBase database ( http://www.microrna.sanger.ac.uk/ ) ( Supplementary Table S3 ). Each reaction was performed in duplicate with a final volume of 20 μl containing 2 μl of the cDNA, 10 μl of 2 × SYBR Green PCR Master mix, of 2 μl and 10 × miScript universal primer and 10 × miScript primer assay. The amplification profile was denaturation at 95 °C, 15 min, followed by 40 cycles of 94 °C, 15 s; 55 °C, 30 s; and 70 °C, 30 s. En face in situ hybridization C57BL/6 mice were killed by CO 2 inhalation and perfused first with saline containing heparin and then with formalin. Aortas were carefully excised, dissected free of surrounding fat tissue, fixed in 4% paraformaldehyde, and tissue samples from LCA and RCA as well as the greater and LC of the aortic arch were taken. For, i n situ hybridization, en face samples were hybridized with 5′,3′-Digoxigenin (DIG)-mmu-miR-712 detection probe (Exiqon) at 60 °C for 18 h, followed by peroxidase-conjugated anti-DIG antibody (Roche). Signal amplification was done by tyramide signal amplification using the Plus cyanine-3 system (TSA-Cy3, PerkinElmer) [52] . Samples were counterstained using DAPI (Sigma) and mounted on glass slides using fluorescence mounting medium (Dako). Samples were imaged using a Zeiss LSM 510 META confocal microscope (Carl Zeiss). Integrated bioinformatics studies We compared a list of putative miR-712 target genes generated by TargetScan [53] to the list of downregulated shear-sensitive genes [1] . The potential target genes were functionally annotated using DAVID [54] ( http://www.david.abcc.ncifcrf.gov ) and enriched onto the Kyoto Encyclopedia of Genes and Genomes (KEGG) pathways [55] to generate a miR-712 interactome. Additional interactions among TIMP3-associated genes were identified through physical protein–protein interaction ( ftp://ftp.ncbi.nih.gov/gene/GeneRIF/ ), transcription factor-target relations [56] and enriched by adding non-mechanosensitive genes with known associations to TIMP3 using Information Hyperlinked over Proteins (iHOP) [57] . Immunohistochemistry Following treatment, ApoE −/− mice were euthanized and perfused with saline containing heparin as described above. LCA and RCA were collected en bloc along with the heart, aortic arch, trachea, oesophagus and surrounding fat tissue. Tissue was embedded in optimal cutting temperature compound (Tissue-Tek), frozen on liquid nitrogen and stored at −80 °C until used. Frozen sections were made starting from the level of the right subclavian artery bifurcation, 300 μm was trimmed away and three sets of 10 consecutive 7 μm thick sections were taken at 300 μm intervals constituting the ‘proximal’ and ‘middle’ portions of the artery. To visualize atherosclerosis development, Oil-red-O staining was carried out using frozen sections using preheated Oil Red O stain at 60 °C for 6 min. The slides were differentiated in 85% propylene glycol for 1 min and rinsed with two changes of distilled water and counterstaining was done using modified Mayer’s haematoxylin for 1 min [10] . Sections were fixed in a 1:1 mixture of methanol/acetone for 10 min at room temperature (RT) and then blocked (1 h, at RT) using 10% (v/v) donkey serum in PBS. Immunohistochemical staining was carried out using following antibodies: versican fragment (1:300) (Abcam), TIMP3 (Abcam) (1:50), VE-cadherin (Santa Cruz) (1:50) and CD45-biotin (eBioscience) (1:100) overnight at 4 °C. Secondary staining for CD45-biotin antibody was performed using streptavidin-conjugated rhodamine red X (Invitrogen), while DyLight 549-conjugated donkey anti-rabbit secondary antibody (Jackson Immunoresearch) (1:250) was used for versican and TIMP3. Samples were imaged using a Zeiss LSM 510 META confocal microscope (Carl Zeiss). Cell culture and shear experiments Immortalized mouse arterial endothelial cells (iMAEC) were generated from C57BL/6 mice. Briefly, aortas from 4-week-old male mice were dissected out and transferred (lumen side down) to a bead of collagen gel consisting of a mixture of type I collagen (Bio-Rad) and EGM2-MV (Lonza) to the final concentration of 1.75 mg ml −1 and were left undisturbed. The explants were observed daily and cultured in incubator in 37 °C and 5% CO 2 . For cell immortalization, cells were incubated with 10 5 neomycin-resistant colony-forming units of the retrovirus vector N-TKmT in 1 ml of complete medium per well in the presence of 8 mg ml −1 polybrene (Sigma). The virus-containing medium was replaced 3 h later with fresh complete medium and G418-resistant cells, were subcultured. All cells were maintained in 10% heat-inactivated fetal bovine serum (Atlanta Biologicals), 100 μM MEM non-essential amino acids, 1% antibiotic-antimycotic (GIBCO) containing DMEM (GIBCO) on 0.1% gelatin-coated 100-mm dishes at 37 °C and 5% CO 2 . For shear experiments, confluent iMAEC in 100 mm dishes were exposed to steady LS (15 dyn cm −2 ), OS (±5 dyn cm −2 ) or static conditions for 24 h using a cone-and-plate shear device for 24 h [58] . Briefly, 100 mm cell culture dishes having confluent iMAEC cells were cultured under LS or OS, while plates at static condition served as controls. Transient transfections with oligonucleotides For the functional tests of miR-712 in vitro , cells were transiently transfected with anti-miR-712 (400 nM; Exiqon), mismatched anti-miR control (400 nM; Exiqon), pre-miR-712 (20 nM; Ambion) or control pre-miR (20 nM; Ambion) using Oligofectamine (Invitrogen), following manufacturer’s protocol as described previously [14] . Cells were sheared for 24 h after transfection. Preparation of whole-cell lysate and immunoblotting Following treatment, cells were washed three times with ice-cold PBS and lysed with 600 μl of RIPA buffer. The protein content of each sample was determined by Bio-Rad DC assay. Aliquots of cell lysate were resolved by size on 10% SDS–polyacrylamide gels and subsequently transferred to a polyvinylidene difluoride membrane (Millipore). The membrane was incubated with the following antibodies: TIMP3 (Abcam; 1:1,000), XRN1 (Abcam; 1:1,000), DGCR8 (Sigma; 1:500), DICER1 (Sigma; 1:1,000), overnight at 4 °C, followed by secondary antibody (Bio-Rad; 1:5,000) for 1 h at RT. Protein expression was detected by a chemiluminescence method. Full sized scans of all western blots are provided in Supplementary Figs S19 and S20 . Isolation of endothelial RNA from mouse aortic arch Aortic arch was harvested from C57BL/6 mice and opened en face . The endothelium was placed against a nitrocellulose membrane soaked in isopropanol for 5 min, and the media and adventitia were peeled away leaving the endothelial monolayer adherent to the nitrocellulose membrane, and RNA was extracted using Qiagen miREasy kit. For each experiment, LC and GC regions from two to four mice were pooled. A panel of markers genes for endothelium (PECAM1), smooth muscle (αSMA) and immune cell (CD11b) was used to determine the enrichment of endothelial RNA from the preparation. Dual-luciferase activity assays Measurement of firefly luciferase activity was obtained at RT using Luc-Pair miR Luciferase Assay Kit (GeneCopoeia) and a single-tube luminometer (Model TD 20/20 Turner Designs, Sunnyvale, CA). Dual-luciferase reporter constructs containing 3′-UTR of TIMP3 with miR-712-binding sites 5′-(G AA GGAA)-3′ (GeneCopoeia) or 3′-UTR of TIMP3 with mutated miR-712-binding site 5′-(G TT GGAA)-3′ (custom cloned at Emory Molecular Biology core facility) were transfected into iMAECs using a Nucleofection Kit (Lonza). iMAECs were transfected first with wild-type or mutated target gene 3′-UTR using HUVEC Nucleofector Kit (Lonza) and were allowed to recover for 24 h. Second transfection was performed using increasing concentrations pre-miR-712 and LNA-anti-miR-712 or respective mismatch controls with Oligofectamine 2000 (Invitrogen). Firefly and Renilla luciferase activities were measured using a Luc-Pair miR Luciferase Assay (GeneCopoeia) as per the manufacturer’s recommendations. Smooth muscle cell proliferation and migration Following anti-miR-712 transfections for 24 h, murine VSMCs were placed in serum-free medium and stimulated with 10 ng ml −1 of platelet-derived growth factor-BB for 24 h and cell proliferation was determined by WST1 assay [59] . To determine migration, VSMCs were transfected with anti-miR-712 or control and were maintained in serum-free media overnight before migration assay. VSMCs were added at a density of 5 × 10 4 cells per well to the upper chamber of a Transwell dish coated with type I rat tail collagen (BD Bioscience) [59] . VSMCs were stimulated with platelet-derived growth factor-BB (10 ng ml −1 ) in the lower chamber. After 4 h, migrated cells were fixed, stained with DAPI and counted from five random fields. Northern blotting Total RNAs were obtained from iMAECs and 25 μg per lane were electrophoresed on 12% denaturating urea gel and transferred onto nitrocellulose membrane. DIG-labelled miR-712 probe (IDT) was used for northern blotting. Anti-DIG antibody conjugated to alkaline phosphatase was used for chemiluminescent detection [60] . 5S rRNA was used as a loading control. Monocyte adhesion assay iMAECs were transfected with pre-miR-712 or control for 24 h and post transfection, leukocyte adhesion assay was performed using 2.5 × 10 5 fluorescent-labelled J774.4 mouse monocyte cells. Adherent cells were quantified by fluorescence microscopy [14] . Endothelial Cell permeability ( in vitro and in vivo ) Cultrex In vitro Angiogenesis Assay Endothelial Cell Invasion Kit was used to determine endothelial permeability using Transfected iMAECs according to manufacturer’s protocol. Fluorescence signals from fluorescein isothiocyanate (FITC)-dextran in the lower chamber were quantified and plotted as arbitrary fluorescence units. For in vivo endothelial permeability assay, 1% Evans blue dye (Sigma) was injected via tail vein (100 μl per animal) 1 week after partial ligation surgery. Animals were killed after 30 min, aortic trees were isolated and imaged by bright field microscopy. Evans blue leakage into the carotids was quantified by NIH Image J software. Soluble-TNFα ELISA iMAECs were treated with TIMP3 expression vector, TIMP3 siRNA, pre-miR-712, anti-miR-712 and their respective controls for 24 h, and then exposed to static or shear conditions for 24 h. s-TNFα in conditioned media was measured using mouse soluble-TNFα enzyme-linked immunosorbent assay kit (R&D Biosystems) following the manufacturer’s protocol. Statistical analyses Statistical analyses were carried out with Graph-Pad Prism (GraphPad Software). All error bars reported are s.e.m. unless otherwise indicated. Pairwise comparisons were performed using one-way Student’s t- tests. Multiple comparisons of means were performed using one-way analysis of variance followed by Tukey’s multiple comparison tests. Differences between groups were considered significant at P -values below 0.05. All miRNA array data were analysed with GenomeStudio software (Illumina). Accession codes: The microarray data have been deposited in NCBI’s Gene Expression Omnibus (GEO) and are accessible through GEO Series accession number GSE52243 . How to cite this article: Son, D. J. et al. The atypical mechanosensitive microRNA-712 derived from pre-ribosomal RNA induces endothelial inflammation and atherosclerosis. Nat. Commun. 4:3000 doi: 10.1038/ncomms4000 (2013).